Ferroelectric polymer networks with high energy density and improved discharged efficiency for dielectric energy storage Ferroelectric polymers are being actively explored as dielectric materials for electrical energy storage applications. However, their high dielectric constants and outstanding energy densities are accompanied by large dielectric loss due to ferroelectric hysteresis and electrical conduction, resulting in poor charge–discharge efficiencies under high electric fields. To address this long-standing problem, here we report the ferroelectric polymer networks exhibiting significantly reduced dielectric loss, superior polarization and greatly improved breakdown strength and reliability, while maintaining their fast discharge capability at a rate of microseconds. These concurrent improvements lead to unprecedented charge–discharge efficiencies and large values of the discharged energy density and also enable the operation of the ferroelectric polymers at elevated temperatures, which clearly outperforms the melt-extruded ferroelectric polymer films that represents the state of the art in dielectric polymers. The simplicity and scalability of the described method further suggest their potential for high energy density capacitors. Dielectric materials capable of controlling charges and storing electrical energy are essential elements in advanced electronics and electrical power systems, ranging from portable electronics and medical defibrillators to hybrid electric vehicles and power grids [1] . Among various dielectric materials, polymers are emerging as the preferred dielectrics for high energy density capacitors owing to their high breakdown strength and graceful failure mechanism [2] , [3] , [4] . In addition, the development of dielectric-polymer-based capacitors has been motivated by the ever-increasing demand for compact, low-cost, lightweight and flexible energy storage devices, since capacitors usually occupy >25% of the volume and weight of devices. Although biaxially oriented polypropylene is currently used as a dielectric in power capacitors because of low dielectric loss and high breakdown strength, its low dielectric constant ( K ~2.2) substantially limits the energy density ( U ) of capacitors (that is, 2–3 J cm −3 at a field of 500 MV m −1 ) [5] . For linear dielectrics, where ε 0 is the vacuum permittivity (=8.85 × 10 −12 F m −1 ) and E is the applied field. An order of magnitude improvement of energy density over that of biaxially oriented polypropylene has been recently achieved in the uniaxially stretched ferroelectric polymers represented by poly(vinylidene fluoride) (PVDF)-based co-polymers [6] . As a result of strong C–F dipoles and spontaneous orientation of dipoles in the crystalline phases, the ferroelectric polymers possess the highest dielectric constant (that is, >12 at a frequency of 1 kHz) at room temperature among the known polymers [7] , [8] , [9] . Unfortunately, the presence of highly coupled dipole interactions and large ferroelectric domains in the ferroelectric polymers results in high energy barriers of switching the dipole direction and strong polarization hysteresis, which in turn incurs high dielectric loss [10] , [11] , [12] . Dielectric loss not only decreases the charge–discharge efficiency and also yields waste heat that reduces the lifetime of capacitors. It has been realized that the size of the ferroelectric domains in PVDF can be altered by disorders or defects in its molecular structure, which mitigate the activation energy of the phase transition [13] . For example, the incorporation of the bulky monomers such as chlorotrifluoroethylene (CTFE) and hexafluoropropylene (HFP) into PVDF main chain gives rise to slimmer polarization loops and enhanced discharged energy densities [6] . Nevertheless, experimental results show that these defects in the PVDF-based co-polymers and terpolymers cannot fully suppress the polarization coupling in the ferroelectric polymers, especially at high electric fields (that is, >10 MV m −1 ). For instance, the dielectric loss as high as ~40% has been found in P(VDF-CTFE) and P(VDF-HFP) films at a field of 300 MV m −1 (refs 13 , 14 ). Furthermore, mechanical stretching, a common practice to improve the mechanical properties and breakdown strength of polymers, simultaneously promotes the conversion of the non-polar to polar phases of ferroelectric polymers, which increases the remnant polarization and polarization hysteresis, and subsequently, results in high ferroelectric loss [15] . In this work, we present a thermal cross-linking approach to tackle the critical issue of energy loss of the ferroelectric polymers under high electric fields. It is found that, in addition to significantly reduced dielectric loss, the resulting networks exhibit many of the ideal features for capacitive energy storage, including improved polarization and markedly enhanced breakdown strength, which leads to high discharged energy densities and great charge–discharge efficiencies of the ferroelectric polymers. Cross-linked ferroelectric polymer networks The cross-linked polymers were prepared by hot-pressing the mixture of P(VDF-CTFE) (15 wt% CTFE), 1,4-bis( t -butyl peroxy) diisopropylbenzene as the initiator and triallyl isocyanurate (TAIC) as the cross-linking agent. It is believed that the Cl groups in P(VDF-CTFE) are abstracted to form macromolecular radicals that are then cross-linked with TAIC [16] ( Supplementary Fig. S1 ). The use of TAIC allows a much higher degree of cross-linking to be achieved than the use of peroxide alone [17] . The cross-linking density measured from equilibrium swelling in cyclohexanone was deliberately varied by adjusting the concentrations of the initiator and TAIC. C1 , C2 and C3 are referred to the cross-linked films containing 1, 3 and 5 wt% initiator, respectively, and 3 wt% TAIC, whose gel contents reach the range of 85–97% ( Supplementary Fig. S2 ). Dynamic mechanical analysis reveals a large increase of storage and loss moduli of the polymers upon cross-linking, for example, from 386.6 and 41.2 MPa of the pristine P(VDF-CTFE) to 811.4 and 123 MPa of C2 , respectively. As shown in Fig. 1a,b , the melting and crystallization points of the cross-linked polymers are found to shift towards lower temperatures, along with smaller enthalpies, relative to the pristine P(VDF-CTFE) in differential scanning calorimetry (DSC) thermographs, indicating that the formation of cross-linking structures hinders the recrystallization [18] . Indeed, as verified in wide-angle X-ray diffraction (WAXD) measurements ( Supplementary Fig. S3 ), the crystal sizes decrease greatly with the introduction of cross-linking structures, for example, from 32 nm at (020) and 19 nm at (110) of the pristine P(VDF-CTFE) to about 24 nm at (020) and 11 nm at (110) of C2 ( Supplementary Fig. S4 ). On the other hand, the degree of crystallinity is only reduced from 34% of P(VDF-CTFE) to 31% of the cross-linked films ( Supplementary Fig. S5 ). It is crucial to retain a substantial degree of crystallinity in the ferroelectric polymers, as their unique dielectric properties are known to originate from the crystalline domains [7] . Moreover, comparison of the Fourier transform infrared spectroscopy (FTIR) spectra of the neat and cross-linked P(VDF-CTFE) films reveals that the chain conformation of the polymers is essentially unchanged upon cross-linking ( Supplementary Fig. S6 ), which is consistent with the WAXD results. The relative fraction of the crystalline phases was quantified using the absorptions at 764 and 840 cm −1 associated with the trans-gauche (TGTG) and all-trans (TTTT) conformation, respectively, as the characteristic peaks for the non-polar α and polar β phase [19] . It is found that the α phase remains as the predominant phase with about 97% content in both pristine and cross-linked P(VDF-CTFE)s. DSC second heating traces of the films are also presented in Fig. 1c . The second heating process in DSC erases the thermal history and provides information on the intrinsic crystalline phase melting of the materials. Unlike the pure P(VDF-CTFE), the Curie transition disappears in the second heating scan of DSC thermographs of the cross-linked polymers, suggesting that the polar phase is destabilized in the cross-linked polymers [20] . A stable non-polar α phase would suppress the remnant polarization and allow for complete transformation from the polar to non-polar phases during discharging cycle, which would lead to improved dipole switchability and reduced ferroelectric hysteresis as illustrated in the following dielectric results. 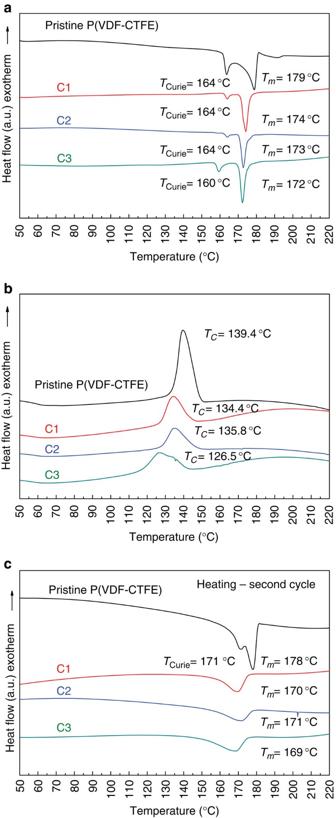Figure 1: Thermal transitions of the P(VDF-CTFE) films. DSC thermographs of pristine and cross-linked P(VDF-CTFE)s collected during (a) the first heating and (b) cooling cycle, and (c) the second heating cycle with a ramp of 10 °C min−1. Figure 1: Thermal transitions of the P(VDF-CTFE) films. DSC thermographs of pristine and cross-linked P(VDF-CTFE)s collected during ( a ) the first heating and ( b ) cooling cycle, and ( c ) the second heating cycle with a ramp of 10 °C min −1 . Full size image Dielectric spectroscopy The frequency dependence of the dielectric constant ( K ) and dielectric loss of the pristine and cross-linked P(VDF-CTFE) is shown in Fig. 2a . The cross-linked polymers exhibit higher K than the un-modified P(VDF-CTFE). For example, C2 gives a K value of ~9.9 at 1 kHz, whereas the value of the un-modified P(VDF-CTFE) is about 9. The improved K can be attributed to smaller crystallite sizes that are more easily switched or aligned under the field. Meanwhile, the lower dielectric loss below 10 kHz of the cross-linked polymers with respect to the pristine P(VDF-CTFE) confirms reduced chain mobility in C1 – 3 as a consequence of cross-linking. 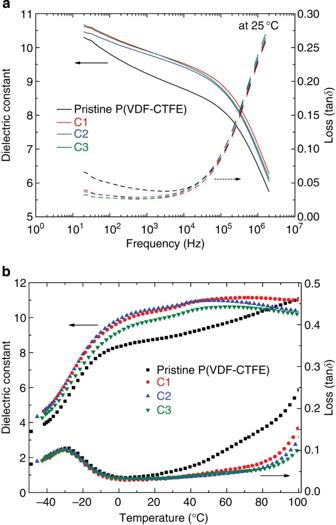Figure 2: Dielectric spectroscopy. Dielectric constant and losses versus (a) frequency measured at 25 °C and (b) temperature measured at 100 Hz with a heating ramp of 10 °C min−1of pristine and cross-linked P(VDF-CTFE) films. Figure 2b illustrates K and loss tangent of the pristine and cross-linked P(VDF-CTFE)s at varied temperatures, where the relaxation peak in the K curve corresponds to the dipolar glass freezing transition of the polymer and a major peak at about −28 °C in the loss spectra arises from the glass transition of the polymer. The appearance of a new dielectric anomaly centred at 45 °C in the K spectra of the cross-linked polymers is ascribed to the relaxation from the polymers located in the cross-linked region, in which cross-linking restricts the chain mobility and thus enhances the activation energy. The observed lower dielectric loss at high temperatures in the cross-linked P(VDF-CTFE)s is a clear indication of substantially reduced space charge conduction, which has further been verified in the high-field dielectric and electrical conductivity measurements (see the results below). Figure 2: Dielectric spectroscopy. Dielectric constant and losses versus ( a ) frequency measured at 25 °C and ( b ) temperature measured at 100 Hz with a heating ramp of 10 °C min −1 of pristine and cross-linked P(VDF-CTFE) films. Full size image Displacement-electric field loop Consistent with the dielectric spectra, the cross-linked films exhibit higher dielectric displacement, for example, 0.064 C m −2 of C1 at 250 MV m −1 , as compared with the neat films (that is, 0.046 C m −2 ) in the displacement–electric field ( D – E ) loop measurements ( Supplementary Fig. S7 ). Even more interestingly, slimmer P–E hysteresis loops are observed in the cross-linked films, denoting lower dielectric loss than that of the unmodified film. 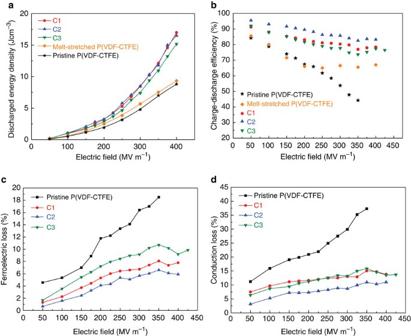Figure 3: High-field dielectric characteristics. (a) Discharged energy density, (b) charge–discharge efficiency, (c) ferroelectric loss and (d) conduction loss of the P(VDF-CTFE) films measured at varied fields. Figure 3a,b show the discharged energy density measured by a modified Sawyer–Tower circuit and the efficiency ( η ) of the charge–discharge cycle as a function of the applied field. The efficiency is given by the ratio of the discharged energy to the stored electric energy, which drops with the applied electric field due to the increase of the dielectric loss. The most significant aspect of the data in Fig. 3b is the radically improved efficiency, especially at high fields, in the cross-linked films. For instance, although the neat and melt-stretched P(VDF-CTFE)s suffer efficiencies that are <40% and 65%, respectively, at 400 MV m −1 , C2 shows an unprecedented efficiency that is around 83%. Consequently, higher discharged energy densities are obtained at relatively low electric fields, for example, discharged energy densities of around 17 J cm −3 are achieved at a field of 400 MV m −1 in C1 – C3 films, which are almost double that of the melt-stretched and pristine P(VDF-CTFE) films with a discharged energy density of ~8-9 J cm −3 (ref. 15 ). Comparatively, an electric field of 600 MV m −1 is needed to achieve the same level of the energy density in the melt-extruded P(VDF-CTFE) and P(VDF-HFP) thin films. Figure 3: High-field dielectric characteristics. ( a ) Discharged energy density, ( b ) charge–discharge efficiency, ( c ) ferroelectric loss and ( d ) conduction loss of the P(VDF-CTFE) films measured at varied fields. Full size image It is also noteworthy that the cross-linking enables the efficient operation of the ferroelectric polymer films at elevated temperatures. For instance, at 70 °C where the melt-stretched P(VDF-CTFE)s normally fails at around 250 MV m −1 with a discharged energy density of 1.6 Jcm −3 , C1 and 2 can still be operated at 400 MV m −1 with discharged energy densities of ~10 J cm −3 ( Supplementary Fig. S8 ). Dielectric loss at high electric fields The dielectric loss of dielectric materials at high electric fields is significantly different from those measured at weak fields because of the emergence of several high-field phenomena. For example, although polypropylenes show negligible loss (≤0.018%) in the dielectric spectra, the loss is as high as ~15% at 600 MV m −1 owing to the exponentially increased leakage current [21] . In addition to high-field conduction, which is a universal phenomenon in all dielectric materials, ferroelectric materials have characteristic ferroelectric switching loss related to polarization hysteresis [11] . To investigate the effect of cross-linking on the different loss mechanisms, the conduction loss is derived from the D – E loops with the assumption that the measured polarization at zero field ( P E =0 ) comes mainly from the leakage current, given that the ferroelectric films in this investigation contain insignificant contents of the polar phase [21] . The relationship between the effective conductivity σ eff and P E =0 can be derived as follows: where T is the period of the applied field. T =1/ f =1/10=0.1 in current case. After σ eff is determined, the conduction loss can be subtracted from the total dielectric loss to give the ferroelectric loss. Figure 3c,d present the ferroelectric and conduction loss of the dielectric films at different electric fields, respectively. Both of the ferroelectric and conduction loss of the pristine (PVDF-CTFE) films increase sharply with the increase of the electric field. On the other hand, significantly reduced ferroelectric loss can be seen in the cross-linked films, for example, 6.6% of C2 versus 18.5% of the pristine P(VDF-CTFE) at 350 MV m −1 , indicating a higher degree of dipole reversibility in the cross-linked films. Concurrently, the conduction loss is reduced remarkably from 37.3% of the neat P(VDF-CTFE) to 10.9% of C2 , which can be rationalized by the formation of deeper traps upon cross-linking. This is corroborated by the shift of the γ L and γ H peaks associated with the characteristics of traps to higher temperatures from the pristine to the cross-linked P(VDF-CTFE)s in the thermally stimulated depolarization current (TSDC) spectra as shown in Fig. 4a (ref. 22 ). The upward shift of β a related to the amorphous relaxation of the glass transition and β c ascribed to molecular motions in the crystalline region manifest the restrained chain mobility in the cross-linked films. The traps reduce the amount of conduction carries and suppress the conductivity. It is evident from Fig. 4b that the resistivity of C2 is more than one order of magnitude lower than that of the neat film, for example, 3.67 × 10 9 Ωm of C2 versus 3.92 × 10 8 Ωm of un-modified P(VDF-CTFE) at 30 MV m −1 . The activation energy estimated from the Arrhenius plot of the conductivity shown in Fig. 4c increases from 1.27 × 10 −19 J of the pristine polymer to 1.6 × 10 −19 J of C2 . 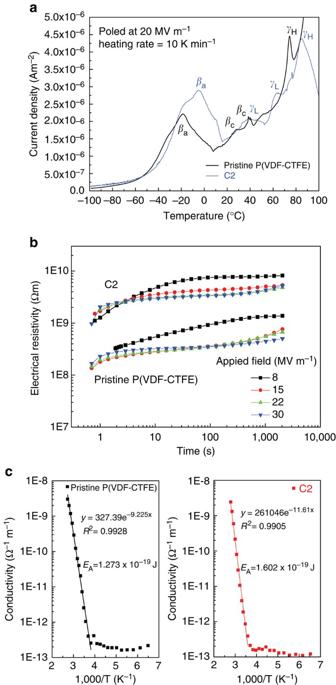Figure 4:Electrical conductivity. (a) TSDC curves, (b) electrical resistivity and (c) Arrhenius plots of electrical conductivity of the P(VDF-CTFE) films. Figure 4: Electrical conductivity . ( a ) TSDC curves, ( b ) electrical resistivity and ( c ) Arrhenius plots of electrical conductivity of the P(VDF-CTFE) films. Full size image Breakdown strength The dielectric strength, which has an exponential effect on the charge storage capacity, is another critical metric of dielectric materials. 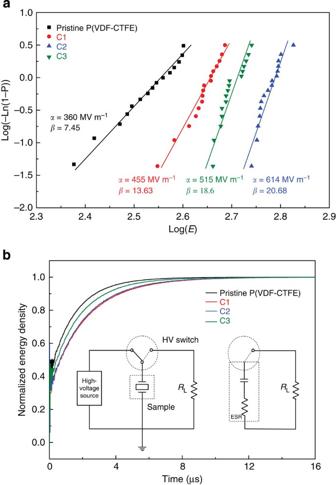Figure 5: Dielectric strength and discharge rate. (a) The Weibull analysis of breakdown strengths, and (b) discharge energy density as a function of time measured from the direct charge of the polymer films to a resistor loadRL=20 kΩ of the pristine and cross-linked P(VDF-CTFE)s. Inset: schematic of the discharge experiment in which the discharged energy density from the sample to aRLwas measured. A high-voltage MOSFET switch is used in the experiment and various losses are treated as an ESR. Figure 5a compares the characteristic breakdown fields of the pristine and cross-linked P(VDF-CTFE)s, where the breakdown results were analysed using a two-parameter Weibull distribution function: Figure 5: Dielectric strength and discharge rate. ( a ) The Weibull analysis of breakdown strengths, and ( b ) discharge energy density as a function of time measured from the direct charge of the polymer films to a resistor load R L =20 kΩ of the pristine and cross-linked P(VDF-CTFE)s. Inset: schematic of the discharge experiment in which the discharged energy density from the sample to a R L was measured. A high-voltage MOSFET switch is used in the experiment and various losses are treated as an ESR. Full size image where P ( E ) is the cumulative probability of electric failure, Ε is the measured breakdown field, α is the characteristic breakdown strength which corresponds to a ~63.2% probability of failure and β is the slope parameter that evaluates the scatter of data [23] . Notably, compared with the breakdown strength of 360 MV m −1 with a β =7.65 for the pristine films, the cross-linked films display greatly improved breakdown strengths and much higher β values. For instance, C2 exhibits a Weibull breakdown strength of 614 MV m −1 , which represents a marked 70% improvement compared with the pristine polymer and is comparable with the melt-stretched P(VDF-CTFE) and P(VDF-HFP) films [15] . Furthermore, a pronounced increase of the β value (for example, β =20.7 for C2 ), suggests a narrow distribution of breakdown strength of the cross-linked films, indicative of excellent dielectric reliability. The decrease in dielectric loss, coupled with the increase in the mechanical properties owing to the incorporation of the three-dimensional networks, all contribute to the improvement in the breakdown strength. Among the cross-linked films, C2 possesses the highest breakdown strength, which is in concert with its lowest dielectric loss. Discharge time One of the unique characteristics of dielectric capacitors compared with other electrical energy storage devices such as batteries is the fast discharge capability. A representative discharge profile from a 20 kΩ load is presented in Fig. 5b , where the discharge time is defined as the time for the discharge energy in a load resistor to reach 95% of the final value. It is found that the cross-linked films release the stored energy at a rate of microseconds, for example, 4.8 μs for C2 , comparable to the pristine films with a discharging time of 3.9 μs. The fitting to the voltage change across the load resistor ( R L ) yields the time constant that is nearly the same as that deduced from R L C , where C is the capacitance. We describe a simple and scalable cross-linking method that enables the ferroelectric polymers to exhibit unprecedented levels of performance for electric energy storage. Although the cross-linked polyethylenes have been commonly used as insulation layer for high-voltage cables because of the improved electric strength [24] , this work has conclusively demonstrated, for the first time, concomitant improvement in the polarization and the reduction of hysteresis of ferroelectric polymers. This is distinctly different from the previous attempts in which the reduction of the hysteresis of the ferroelectric polymers is usually achieved at the expense of polarization. For example, although P(VDF-CTFE) enjoys a much narrower D – E loop than PVDF, the maximum displacement is reduced from 0.07 to 0.049 C m −2 at 300 MV m −1 with the introduction of bulky CTFE into PVDF [25] . Previously, it has been reported that reduction of the hysteresis can be obtained in electron-irradiated ferroelectric polymers [26] . However, ionizing radiation decreases the crystallinity and the maximum polarization, as well as introduces the ionic species into the crystalline phases to yield high leakage current. Reduced maximum polarization has been found in the cross-linked poly(vinylidene fluoride-trifluoroethylene) (PVDF-TrFE) possible due to greatly impaired crystallinity [27] , [28] . The introduction of deep traps upon cross-linking as confirmed in the TSDC spectra are responsible for the observed dramatic decrease in conduction loss. Besides the reduced crystal size, it is postulated that the cross-linking networks also render elasticity to pull the poled polar conformation back to the non-polar conformation during discharging, which enhances the reversibility of crystalline dipoles for reduced hysteresis, and accordingly, low ferroelectric switching loss. The enhancement of dipole reversibility has been further confirmed by the significantly lower ratios of remnant polarization versus maximum polarization shown in the cross-linked films than those of the pristine P(VDF-CTFE)s as shown in Fig. 6 . C2 has the smallest ratio of remnant/maximum displacement, consistent with its lowest ferroelectric loss among the cross-linked films. It is interesting to note that C3 has a higher ferroelectric loss and higher ratio of remnant/maximum displacement than C1 – C2 , although it has the smallest crystallite sizes. We speculate that highly cross-linking structures in C3 may impede the oriented dipoles in the amorphous phase of P(VDF-CTFE) to be reverted to an antiferroelectric-like or random state at a zero electric field during the discharge process, which subsequently decreases the released energy density and the charge–discharge efficiency. 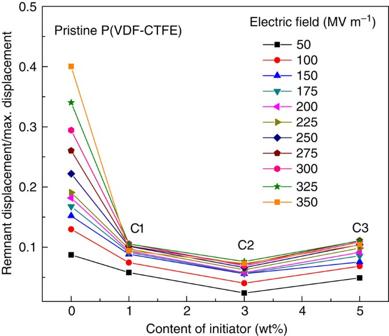Figure 6: Evaluation of dipole reversibility. Ratio of the remnant and maximum displacements of pristine and cross-linked P(VDF-CTFE)s. Figure 6: Evaluation of dipole reversibility. Ratio of the remnant and maximum displacements of pristine and cross-linked P(VDF-CTFE)s. Full size image In conclusion, compared with the mechanically stretched ferroelectric polymer films, the cross-linked polymers posses the same level of remarkable breakdown strength and confer superior dielectric properties at high electric fields, including lower loss, higher charge–discharge efficiencies, superior energy densities and improved elevated temperature performance. For instance, a discharged energy density of 17 J cm −3 with a charge–discharge efficiency of ~83% is obtained in the cross-linked films at 400 MV m −1 , which is more than two times higher that of the melt-stretched P(VDF-CTFE) films with an efficiency <65% that represents the state-of-the-art dielectric polymers. We thus expect this work to open up a new avenue to boost the performance of ferroelectric polymers for high energy density capacitors. Materials preparation P(VDF-CTFE) was supplied by Solvay (Solef 31508). 1,4-Bis( t -butyl peroxy) diisopropylbenzene and TAIC were purchased from Herculese and Aldrich, respectively. All materials were used as received. The compounds were mixed in a Model 6770 Freezer Miller (SPEX) and then pressed at 200 °C and 4,000 psi pressure for 2 h followed by ice-water and air quenching. The typical film thickness is around 15 μm. Characterization The gel contents and cross-link densities were examined using the ASTM D2765-01 standard procedure. The thermal transition data were obtained by TA Instruments Q100 differential scanning calorimeter at a heating/cooling ramp of 10 °C min −1 in nitrogen atmosphere. WAXD studies were conducted using a Scintag Cu-KR diffractometer with an X-ray wavelength of 1.54 Å and the data were deconvoluted using ‘Peakfit’ software with a Gaussian–Lorentz superposition fitting functions. FTIR spectra were obtained in the attenuated total reflectance mode using ZnSe crystal as a contact to the samples on Varian Digilab FTS-8010 spectrometer at room temperature. Gold electrodes of a typical thickness of 60 nm were sputtered on both sides of the polymer films for the electrical measurements. Dielectric constant and loss were measured using an Agilent LCR meter (E4980A). Dielectric spectra were acquired over a broad frequency (10–10 6 Hz) and temperature (−40–100 °C) using a Hewlett Packard 4284A LCR meter in conjunction with a Delta Design oven model 2300. High-field D – E loops were collected using a modified Sawyer–Tower circuit, where the samples were subjected to a triangular unipolar wave with a frequency of 10 Hz. Dielectric breakdown strength measurements were performed on a TREK P0621P instrument using the electrostatic pull-down method under a dc voltage ramp of 500 V s −1 . TSDC spectra and electrical conductivity were measured using Hewlett Packard 4140B pA meter with Kepco BOP1000M as a high-voltage source and performed in a Delta Design oven model 2300. Measurement of gel content The analysis was performed by solvent swelling and extraction of samples in cyclohexanone (boiling point 156 °C) heated to reflux for 12 h (ASTM D2765). The insoluble component was recovered and immediate weighed to give the weight of the swollen gel at solvent equilibrium. The gels were then dried at 80 °C in vacuum to give the dry weight of the insoluble component. The gel contents were then simply a fraction of dry insoluble weight to the initial weight. The average molecular weight between two adjacent cross-linked sites was calculated using Flory–Rehner swelling theories [17] where M c is the average molecular weight between cross-links; V pol =1/(1+( f −1) ( ρ pol / ρ sol )); f is the swelling factor and equal to the ratio of weight of the swollen gel to dry gel; ρ pol is the density of P(VDF-CTFE) (that is, 1.79 gcm −3 ); ρ sol is the density of cyclohexanone (that is, 0.97 gcm −3 ); μ is the Huggins solvent–polymer interaction parameters (that is, −0.3 for P(VDF-CTFE)) and V o is the molar volume of cyclohexanone (that is, 139.3 cm 3 mol −1 ). Calculation of the fractions of the crystalline phases The fraction of the β crystalline phase present in each sample was calculated by using where X α and X β are the mass fractions of the α and β crystalline phases, A α and A β are the FTIR absorption bands (peak heights) at 764 and 840 cm −1 , respectively, and 1.26 is the ratio of absorption coefficients at 764 and 840 cm −1 . Discharge experiments The discharged energy density was measured by the modified Sawyer–Tower circuit [29] . In the fast discharge experiment, the polymer film capacitor was charged to a given field E and through a high-voltage MOSFET switch (Behlke HTS81), the stored energy was discharged to a resistor R L as schematically shown in inset of Fig. 5b . R L can be varied so that the discharge behaviour of the polymer film capacitor can be characterized over a broad time domain. In dielectric materials, there exist various losses which can be treated as an equivalent series resistor (ESR) as illustrated in inset of Fig. 5b . Therefore, the total discharged energy U e to the load resistor R L is smaller than the total stored energy U 0 . However, if R L >>ESR, U e will be close to U 0 . For the discharge experiment performed here, an ESR can be introduced to link the total discharged U e to the total stored energy density U 0 In general, ESR will also depend on the discharge speed (or R L ). In the frequency domain analysis, where tan δ is the dielectric loss, ω is the angular frequency and C is the capacitance. For the dielectric polymers investigated here, ESR( ω ) in equation 7 decreases with frequency. Consequently, at the initial time of discharging (high frequencies) to R L in which most of the energy is released, ESR effect is small. The influence of ESR increases at later stage (longer time and lower frequencies) of discharging process. How to cite this article: Khanchaitit, P. et al. Ferroelectric polymer networks with high energy density and improved discharged efficiency for dielectric energy storage. Nat. Commun. 4:2845 doi: 10.1038/ncomms3845 (2013).